AtNIGT1/HRS1 integrates nitrate and phosphate signals at theArabidopsisroot tip Nitrogen and phosphorus are among the most widely used fertilizers worldwide. Nitrate (NO 3 − ) and phosphate (PO 4 3− ) are also signalling molecules whose respective transduction pathways are being intensively studied. However, plants are continuously challenged with combined nutritional deficiencies, yet very little is known about how these signalling pathways are integrated. Here we report the identification of a highly NO 3 − -inducible NRT1.1-controlled GARP transcription factor, HRS1, document its genome-wide transcriptional targets, and validate its cis -regulatory elements. We demonstrate that this transcription factor and a close homologue repress the primary root growth in response to P deficiency conditions, but only when NO 3 − is present. This system defines a molecular logic gate integrating P and N signals. We propose that NO 3 − and P signalling converge via double transcriptional and post-transcriptional control of the same protein, HRS1. As sessile organisms, plants have evolved a myriad of adaptive mechanisms to cope with nutritional limitations in their environment. In particular, plants adapt their root development differently according to nutritional cues [1] . Nitrate (NO 3 − ) and phosphate (PO 4 3− ), two major phyto-macronutrients, are also well known signalling molecules shaping root development through partly defined molecular pathways [2] , [3] , [4] , [5] , [6] . For the inorganic phosphate (Pi) response, prd [7] , lpr1, lpr2 (ref. 8 ) , pdr2 (refs 9 , 10 ) , phr1 (refs 11 , 12 ) and siz1 (ref. 13 ) mutations have been found to affect the primary root growth. Concerning NO 3 − , its effect is more related to lateral root growth, with the implication of several molecular actors (thoroughly reviewed in refs 4 , 14 ), and has been shown to counteract the effect of glutamate on the primary root growth [15] . Despite this knowledge, a mechanism by which a plant integrates the presence or the absence of combinations of such key nutritional molecules is still largely unknown. Recently, the NLA (nitrogen limitation adaptation) and PHO2 proteins (two ubiquitin ligases) were found to control PO 4 3− transporter trafficking (PHT1 family), which results in a nitrogen-dependent PO 4 3− accumulation in leaves [16] , [17] , [18] , [19] . Despite these first hints into the molecular connections between P and N nutrition, nothing has so far been revealed concerning the mechanisms by which NO 3 − affects PHO2 or NLA activities. The root tip is known to be at the forefront of Pi sensing [8] . It is also the territory of expression of the recently identified nitrate sensor NRT1.1 (refs 20 , 21 ). Thus, it represents the perfect place for such nutritional signalling interactions. The present work reports such missing mechanism. Here we show that HRS1 and HHO1 are two early NO 3 − -regulated transcription factors (TFs). We document genome-wide HRS1 direct targets and demonstrate that hrs1;hho1 double mutant is involved in the primary root growth repression in response to a combination of N and P signals. We report a potential mechanism to explain this phenotype as HRS1 is under a dual transcriptional and post-transcriptional control. Finally, an in planta genome-wide investigation provides potential signalling pathways under HRS1 and HHO1 influence. Identification of two NO 3 − -regulated TFs A set of early nitrate-regulated gene clusters have been previously identified in a genome-wide investigation [22] . Among these, At1g13300 was one of the most rapidly and strongly upregulated TFs (with a significant response recorded within 6 min after treatment). The early and marked induction of At1g13300 and several genes involved in the nitrate uptake and assimilation have been confirmed in an independent set of experiments ( Fig. 1 ). In roots, NO 3 − provision triggers the induction of the two sentinel gene transcripts ( NIR and NRT2.1 ) after 10 and 30 min respectively. This validates the conditions of the N treatment ( Fig. 1a ). As predicted by the previous experiments, At1g13300 accumulation was rapidly and strongly upregulated (10-fold within 10 min) compared with the KCl mock treatment ( Fig. 1a ). These observations are consistent with the previous reports corresponding to genome-wide or specific reverse transcription quantitative (qPCR) investigations [6] , [23] , [24] , [25] . 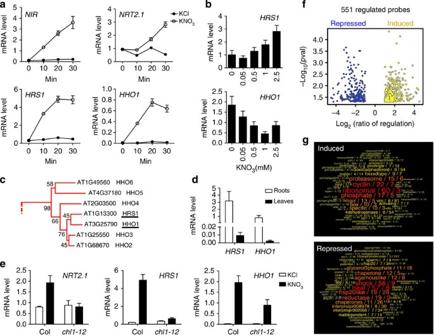Figure 1:HRS1andHHO1are twoArabidopsistranscription factors highly induced by NO3−downstream the nitrate sensor activity. Identification of HRS1 direct targets. (a) Dynamic nitrate response of mRNA forNIR,NRT2.1(NO3−responsive sentinels),HRS1(At1g13300) andHHO1(At3g25790) in roots of 14-day-old seedlings treated with 1 mM KNO3or 1 mM KCl (as mock treatment), values are means±s.e.m. (n=4). (b) Steady-state level of HRS1 and HHO1 mRNA in roots of plants grown for 14 days on solid media containing 0.5 mM KH2PO4and different KNO3concentrations, values are means±s.e.m. (n=4). (c) A subfamily of the G2-like transcription factors phylogenetic tree built by ClustalW alignment and maximum likelihood method, values are bootstraps based on 500 replicates (seeSupplementary Fig. 1). (d) HRS1 and HHO1 mRNA levels in roots and leaves of WT plants grown for 14 days on basal MS media containing 0.5 mM KH2PO4and 2.5 mM KNO3, values are means±s.e.m. (n=3). (e)HRS1andHHO1nitrate induction is affected in roots ofchl1-12mutant mutated in NRT1.1. WT andchl1-1214-day-old seedlings were treated for 30 min with 1 mM KNO3or 1 mM KCl (as mock treatment). All transcript levels were quantified by reverse transcription qPCR and normalized to two housekeeping genes (ACT and CLA), values are means±s.e.m. (n=4). (f) Volcano plot of HRS1 direct regulated targets identified by TARGET (transient assay reporting genome-wide effects of transcription factors) procedure36. (g) Semantic gene enrichment analysis results showing overrepresented terms in the list of the HRS1 direct up- and downregulated genes. Figure 1: HRS1 and HHO1 are two Arabidopsis transcription factors highly induced by NO 3 − downstream the nitrate sensor activity. Identification of HRS1 direct targets. ( a ) Dynamic nitrate response of mRNA for NIR , NRT2.1 (NO 3 − responsive sentinels), HRS1 (At1g13300) and HHO1 (At3g25790) in roots of 14-day-old seedlings treated with 1 mM KNO 3 or 1 mM KCl (as mock treatment), values are means±s.e.m. ( n =4). ( b ) Steady-state level of HRS1 and HHO1 mRNA in roots of plants grown for 14 days on solid media containing 0.5 mM KH 2 PO 4 and different KNO 3 concentrations, values are means±s.e.m. ( n =4). ( c ) A subfamily of the G2-like transcription factors phylogenetic tree built by ClustalW alignment and maximum likelihood method, values are bootstraps based on 500 replicates (see Supplementary Fig. 1 ). ( d ) HRS1 and HHO1 mRNA levels in roots and leaves of WT plants grown for 14 days on basal MS media containing 0.5 mM KH 2 PO 4 and 2.5 mM KNO 3 , values are means±s.e.m. ( n =3). ( e ) HRS1 and HHO1 nitrate induction is affected in roots of chl1-12 mutant mutated in NRT1.1. WT and chl1-12 14-day-old seedlings were treated for 30 min with 1 mM KNO 3 or 1 mM KCl (as mock treatment). All transcript levels were quantified by reverse transcription qPCR and normalized to two housekeeping genes (ACT and CLA), values are means±s.e.m. ( n =4). ( f ) Volcano plot of HRS1 direct regulated targets identified by TARGET (transient assay reporting genome-wide effects of transcription factors) procedure [36] . ( g ) Semantic gene enrichment analysis results showing overrepresented terms in the list of the HRS1 direct up- and downregulated genes. Full size image The At1g13300 gene encodes a myb-related TF belonging to the GARP (GOLDEN2, ARR-B, Psr1) family; a homologue to NIGT1 identified in rice [26] . The GOLDEN2-like subgroup is composed of 40 protein sequences (AGRIS, http://arabidopsis.med.ohio-state.edu/ ). It encompasses proteins involved in various processes ranging from the control of chloroplast and leaf development (GLKs [27] and KANADIs [28] ) to nutritional reprogramming in plants (PHR1 and PHL1 (ref. 12 )). A phylogenetic tree has been built out of the 40 G2-like protein sequences ( Supplementary Fig. 1 , see Methods). It shows that At1g13300 belongs to a small group of seven proteins sharing high sequence similarity to each other, but quite well separated from the rest of the tree ( Fig. 1c ; Supplementary Fig. 1 ). This sub-group within the larger GARP family has already been reported on its own [29] . We thus kept the proposed nomenclature and extended the relationships between the other members of the GARP family. At1g13300 is named HRS1 (hypersensitive to low Pi-elicited primary root shortening 1) [29] . HRS1 is a paralogue with its closest neighbour, At3g25790, which has been named HHO1 (HRS1 homologue 1) [29] . It is noteworthy that these two close homologues, HRS1 and HHO1, have recently been identified among the 2,594 gene pairs that were defined in an effort to isolate redundant duplicated genes [30] . Interestingly, HHO1 showed a similar pattern of expression to HRS1 with a strong upregulation (>50-fold) within the first 20 min of nitrate treatment ( Fig. 1a ), both being mainly expressed in roots ( Fig. 1d ). Furthermore, HRS1 and HHO1 messenger RNA (mRNA) levels in roots are dependent on nitrate concentration in the media. Wild Type seedlings constantly grown for 14 days on media containing increasing NO 3 − concentrations presented a gradual transcriptional response of HRS1 and HHO1 ( Fig. 1b ). Interestingly, despite the fact that both genes are upregulated by NO 3 − provision, the increasing KNO 3 concentration has opposite effects on their steady-state expression levels: HRS1 is positively regulated and HHO1 is negatively affected ( Fig. 1b ). In conclusion, HRS1 and HHO1 are two root-specific, NO 3 − -controlled TFs (found to be responsive in the nitrate reductase-null mutant in previous genome-wide investigations [31] ). A meta-analysis [6] also demonstrated that HRS1 and HHO1 are under the control of NRT1.1 protein activity. Indeed, their nitrate induction is strongly and robustly affected in chl1 mutants (defective in the NRT1 .1 gene) in two independent transcriptomic data sets issued from two independent laboratories [25] , [32] . We also performed analysis in our conditions and indeed recorded defects in nitrate responsiveness in an independent chl1 deletion allele of NRT1.1 ( chl1-12 ; Fig. 1e ). In the chl1-12 mutant, the 24-fold induction (after 30 min of NO 3 − treatment) of HRS1 expression is totally abolished and the HHO1 strong induction (~100-fold) is reduced to a third. Finally, HRS1 and HHO1 are also under the influence of NLP genes (NIN-like TFs) implicated in N-signalling [33] , and are found to be bound (assayed by chromatin immunoprecipitation sequencing) by NLP7 (ref. 34 ). Collectively, these results demonstrate that the TF paralogues, HRS1 and HHO1 are each strongly NO 3 − controlled (for example, are among the most, if not the most, robustly NO 3 − -regulated genes in many data sets [35] ) and positioned downstream of the early regulators NRT1.1/CHL1 and NLP7-6 activity. Identification of HRS1 direct targets At the outset of this study nothing was known about the molecular mechanism downstream of At1g13300 (HRS1). We thus decided to investigate the genome-wide effect of this TF using a transient assay system for TF perturbation that can uncover direct targets only [36] . Indeed, we have shown for other TFs (ABI3 and bZIP1) that using this system to uncover the direct regulated targets of a TF can give very important clues about its functional role in planta [36] , [37] . We thus speculated that we could retrieve the functional in planta activity of At1g13300 by studying the set of its direct targets. To search for such genes that are directly regulated by At1g13300, we used the TARGET (Transient Assay Reporting Genome-wide Effects of Transcription factors) approach described by Bargmann et al. [36] Briefly, protoplasts are isolated from roots of 10-day-old Arabidopsis seedlings and transformed with the plasmid pBeaconRFP_GR-HRS1, expressing a translational fusion (N-ter) between HRS1 and the rat glucocorticoid receptor (GR) under the control of the pCaMV35S promoter. Protoplasts are treated with (i) dexamethasone (DEX; triggers GR–TF fusion entrance in the nucleus) and (ii) cycloheximide (CHX; translation inhibitor that prevents activation of indirect targets) [36] . Because of the possibility that HRS1 acts as a part of a NO 3 − -regulated protein complex (as it is itself NO 3 − regulated, see above), we kept NO 3 − present during the whole TARGET procedure. After fluorescent-activated cell sorting selection (based on red fluorescent protein signal provided by an independent cassette in the plasmid) of transformed protoplasts, total RNA was isolated from GR–HRS1 protoplasts and used for the transcriptomic analysis. The statistical analysis (see Methods) of transcriptome results identified 551 gene probes whose expression was affected by GR-HRS1 nuclear import. The corresponding genes were classified as up- and downregulated HRS1 direct target genes ( Fig. 1f ; Supplementary Data 1 ). To search for the functions that are globally affected by HRS1 activity, we performed two kinds of analysis. First, we determined over-represented gene ontology (GO) categories using the VirtualPlant and agriGO platforms [38] , [39] . Second, we developed our own algorithm that search for over-represented terms in a set of TAIR v10 gene description (see Methods). Both approaches yielded very similar conclusions: At1g13300 (HRS1) collectively induces genes related to ‘ phosphate ’ and ‘ cell division ’ (including the terms meristematic activity, cyclin and ribosomal proteins ). On the other hand, in the list of HRS1 downregulated genes, the most frequent terms were ‘ heat ’ ‘ shock ’ and the most represented functions were linked to response to stresses ( Fig. 1g ; Supplementary Data 1 ; Supplementary Fig. 6 ). This genome-wide investigation of the At1g13300 HRS1 TF direct targets brought us to be interested in the interaction between NO 3 − signalling (that controls transcriptional activation of this gene) and P nutrition that seems to be one of the functions under its influence [29] . Taken together with the fact that HRS1 belongs to the same TF family as the very well characterized PHR1 gene [11] , [12] , known to be central in the control of P starvation response, we decided to employ a reverse genetic approach to understand the role of HRS1 in the control of NO 3 − and Pi signalling interactions. HRS1 and HHO1 repress primary root growth The hrs1-1 mutant was obtained from ABRC seeds stock center, and the T-DNA insertion and the absence of HRS1 full-length transcripts were confirmed ( Supplementary Fig. 2 ). First, we tested the growth of the hrs1-1 mutant on different media containing +P (0.5 mM KH 2 PO 4 ) or −P combined with different NO 3 − concentrations (0, 0.05, 0.5, 1 and 2.5 mM). The results did not lead to any reliable/robust phenotype ( Supplementary Fig. 3a ), as previously reported [29] . We thus hypothesized that this could be due to functional redundancy of the two NO 3 − -induced close relatives HRS1 and HHO1 ( Fig. 1c ). We thus tested the double mutant hrs1-1;hho1-1 (see molecular characterization in Supplementary Fig. 2 ) on the same P/N varying conditions. As previously shown [8] , the primary root growth of WT plants was impaired on −P conditions. Interestingly, however, the primary root growth of the double hrs1;hho1 mutant was strongly insensitive to the −P conditions ( Fig. 2a,b ). This insensitivity is also manifested on transfer experiments ( Supplementary Fig. 3b,c ). The fact that the hsr1;hho1 double mutant is resistant to −P conditions complements previous observations reporting that the overexpression of HRS1 indeed confers hypersensitivity to low P conditions [29] . More importantly, NO 3 − is required for the manifestation of the hrs1;hho1 double mutant phenotype. Indeed, the phenotype of the hrs1;hho1 double mutant is lost in plants grown on −N/−P conditions. More precisely, the presence of at least 0.05 mM NO 3 − in the media was necessary for the appearance of the root phenotype in response to Pi-depleted conditions ( Fig. 2c ). These results suggest that the HRS1 and HHO1 proteins act as repressors of primary root development specifically when PO 4 3− is absent and NO 3 − is present in the media. It is thus tempting to propose that the well-known primary root growth repression in response to low P conditions is an active process that is influenced by (i) NO 3 − and (ii) the NO 3 − -regulated TFs HRS1 and HHO1. 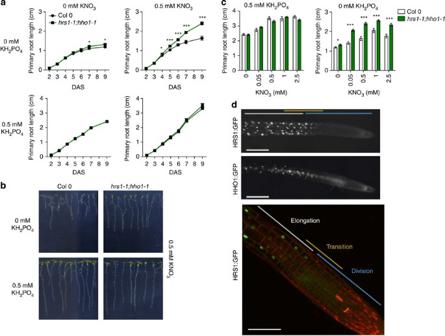Figure 2: HRS1 and HHO1 are two nuclear factors expressed in meristematic elongating cells repressing root growth in response to combination of P and N availability. (a) Primary root growth measurement over time of Col andhrs1-1;hho1-1seedlings grown on P/N combinations. In +P/−N conditions, the WT and mutant slopes overlap. (b) Nine-day-old seedlings grown on 0.5 mM of NO3−and PO43−under different conditions (0–0.5 mM added). (c) Effect of different nitrate concentrations in the media on the primary root growth ofhrs1-1;hho1-19 day-old seedlings. Values represent the means±s.e.m. (n=30). Asterisks indicate significant differences from WT plants (*P<0.05; ***P<0.001; Student’st-test). (d) Epifluorescent and confocal imaging of pHRS1:HRS1:GFP and pHHO1:HHO1:GFP expressing plants (scale bars, 200 μm). Figure 2: HRS1 and HHO1 are two nuclear factors expressed in meristematic elongating cells repressing root growth in response to combination of P and N availability. ( a ) Primary root growth measurement over time of Col and hrs1-1;hho1-1 seedlings grown on P/N combinations. In +P/−N conditions, the WT and mutant slopes overlap. ( b ) Nine-day-old seedlings grown on 0.5 mM of NO 3 − and PO 4 3− under different conditions (0–0.5 mM added). ( c ) Effect of different nitrate concentrations in the media on the primary root growth of hrs1-1;hho1-1 9 day-old seedlings. Values represent the means±s.e.m. ( n =30). Asterisks indicate significant differences from WT plants (* P <0.05; *** P <0.001; Student’s t -test). ( d ) Epifluorescent and confocal imaging of pHRS1:HRS1:GFP and pHHO1:HHO1:GFP expressing plants (scale bars, 200 μm). Full size image HRS1 and HHO1 are expressed in elongating root cell nuclei To further investigate the in planta roles of the HRS1 and HHO1 proteins, we constructed native promoter gene green fluorescent protein (GFP) lines for these two TFs. Epifluorescence and confocal imaging of transgenic pHRS1:HRS1:GFP and pHHO1:HHO1:GFP plants indicate that the two proteins are expressed and localized in the nucleus of epidermal and cortex cells in elongating roots ( Fig. 2d ; Supplementary Fig. 4 ). HRS1 and HHO1 expression is found in the transition domain of the root apical meristem and in the elongation zone ( Fig. 2d ). The expression of HRS1 was also visible in root hair cells ( Supplementary Fig. 4 ). The localization of these two proteins supports the idea that HRS1 and HHO1 are nuclear-localized TFs involved in the control of the root elongation. HRS1 binds to two different cis -regulatory elements To identify cis -regulatory elements (CREs) directly targeted by HRS1 protein, we searched for conserved motifs in the promoters of the most strongly up- and down-regulated target genes. Thus, we examined the 500 bp promoter sequences upstream the transcription start site for the 120 top induced and repressed genes (based on fold regulation upon DEX treatment) from the TARGET transcriptome analysis (presented in Fig. 1f ). Five strongly significant motifs were retrieved using the MEME algorithm [40] . The two cis -motifs, which were over-represented in the promoters of genes upregulated by HRS1, display the consensus sequences AGANNNAAA and AAACNNAACC. By contrast, the HRS1 downregulated genes share three over represented motifs: AANNAGA, TGGGC and GAGA ( Fig. 3a ). Among these last three cis -motifs, the TGGGC(C/T) motif was already known as the core-binding sequence of the CRE for TCP (teosinte branched1, cycloidea, PCF) TFs [41] . Inspired by the consensus sequences above, we defined five motifs (M1–M5; Supplementary Fig. 5c ; Supplementary Table 1 ) that were tested in vitro for direct binding by HRS1 in Electophoretic Mobility Shift Assays (EMSAs). The HRS1 recombinant protein produced a shift for motifs #1, 2, 3 and 5. The shifts were completely reverted by the competition of a 200-fold molar excess of the same unlabelled probe ( Supplementary Fig. 5d ). No band shift was detected for motif #4, which corresponds to the TCP-binding site. This means that TCP TFs may be partners of HRS1 mediating its repressive transcriptional activity. Motifs #1, 2 and 3 in the HRS1-induced genes share the core sequence AGA and the motif #5 the core AACC (already known as part of the GLK1/2-binding site [27] ). This is in accordance with the recent finding that a particular TF can bind to distinct cis -elements [42] . The specificity of HRS1 binding to the selected DNA probes was confirmed by EMSA analysis, using unlabelled probes mutated on the above described core sequences (AGA and AACC). Ten-, 25-, and 50-fold molar excess of unlabelled mutant probes could not compete with HRS1 binding to motifs #1, 3 and 5, thus confirming that HRS1 binding is maintained by AGA and AACC core sequences ( Supplementary Fig. 5e ). 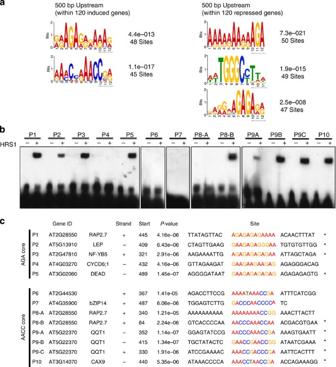Figure 3: Identification ofcis-regulatory elements and binding of HRS1 to the promoters of ‘meristem-related’ genes. (a) Weight matrix representation of the motifs retrieved by the MEME algorithm analysis from the 500 bp sequences upstream the transcription start sites of the top 120 direct up- and downregulated HRS1-target genes. (b) EMSA analysis on 30-bp promoter fragment from HRS1 directly regulated genes (from TARGET analysis); biotin-labelled DNA probes (20 fmol), HRS1–GST protein (50 ng). (c) List of the promoter fragments sequences used for EMSA analysis ina. For each promoter the gene ID, the common name and the strand position is indicated. Figure 3: Identification of cis -regulatory elements and binding of HRS1 to the promoters of ‘ meristem-related ’ genes. ( a ) Weight matrix representation of the motifs retrieved by the MEME algorithm analysis from the 500 bp sequences upstream the transcription start sites of the top 120 direct up- and downregulated HRS1-target genes. ( b ) EMSA analysis on 30-bp promoter fragment from HRS1 directly regulated genes (from TARGET analysis); biotin-labelled DNA probes (20 fmol), HRS1–GST protein (50 ng). ( c ) List of the promoter fragments sequences used for EMSA analysis in a . For each promoter the gene ID, the common name and the strand position is indicated. Full size image To obtain functional explanations of the root developmental phenotype described ( Fig. 2a–c ), we tested whether HRS1 was also able to bind native CREs found in promoters of genes categorized as ‘ meristem-related ’ genes. For that we used 30-bp promoter fragments as EMSA probes. HRS1 produced a significant shift for 9 of 13 promoter fragments tested ( Fig. 3b,c ). Promoters have been selected as they are; (i) induced by HRS1 in the TARGET system ( Fig. 1f ); and (ii) they are classified by GO as being involved in meristematic activity . To summarize, HRS1 is shown to be able to bind the promoter sequences of RAP2-7 (related to AP2.7; AT2G28550 ), LEP (leafy petiole; AT5G13910 ), the NF-YB5 (nuclear factor Y, subunit B5; AT2G47810 ) TF, the helicase DEAD ( AT3G02060 ), the DNA-binding protein QQT1 (quatre quart 1; AT5G22370 ) involved in embryo development, and the cation calcium exchanger CAX9 (cation calcium exchanger 9; AT3G14070 ). These results show that HRS1 possesses two distinct target CREs found in HRS1-activated genes belonging to developmental processes pathways. HRS1 is post-transcriptionally controlled by P provision Since HRS1 is clearly strongly transcriptionally activated by the NO 3 − signalling pathway ( Fig. 1a ), and it is involved in the convergence of Pi and NO 3 − signals ( Fig. 2 ), we investigated how Pi and NO 3 − might affect the levels of HRS1 protein. As expected for such a NO 3 − -induced transcript ( Fig. 1 ), the HRS1 protein strongly accumulates in response to NO 3 − treatment ( Fig. 4a ). Interestingly, in whole roots, HRS1:GFP protein accumulation was reduced after 24 and 48 h of Pi deprivation ( Fig. 4b ). In the same conditions (48-h Pi starvation), HRS1 mRNA levels are not changed, even if the plant felt the Pi deprivation (as reported by IPS1 , Fig. 4b ). These findings suggest a possible post-transcriptional regulation of HRS1 by Pi provision. Interestingly, this interaction of NO 3 − transcriptional induction of HRS1, together with its post-transcriptional regulation in response to −P, could constitute a mechanism that entangles both nutritional signals. To confirm this hypothesis, the NO 3 − transcriptional regulation has to be conserved independent of the preceding P treatment. To demonstrate this, we verified that the transcriptional regulation of HRS1 by NO 3 − is maintained in P varying conditions ( Fig. 4c ). Furthermore, we observed that the accumulation of the HRS1 protein accumulation is not affected by P provision in the short-term experiments. This demonstrates that NO 3 − and −P signals act early (within minutes) and late (within days) at the transcriptional and post-transcriptional levels, respectively ( Fig. 4 ). To delve further into one potential mechanism of the P effect on HRS1 activity, we analysed HRS1–GFP protein half-life in P varying conditions ( Fig. 5a,b ). We recorded that −P treatment shifts the HRS1 half-life from ~20 to 30 min. Interestingly, this mechanism is not restricted to HRS1, since another nitrate-regulated protein is under this kind of regulation ( Fig. 5c ). Indeed, we have found that the nitrate transporter/sensor NRT1.1 is strongly destabilized on −P conditions (as compared with another membrane protein PIP2.1, Fig. 5c ). This demonstrates that P deficiency conditions may broadly affect nitrate-regulated proteins to convey a layer of the NO 3 − and PO 4 3− signal interaction. 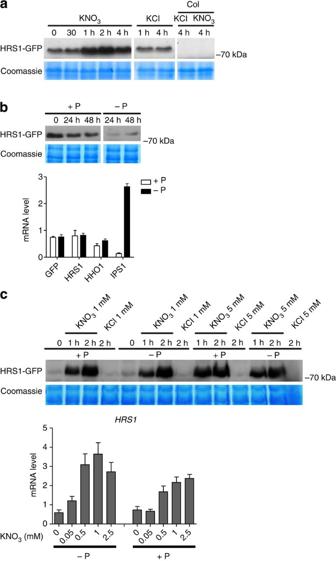Figure 4: P and NO3−provisions influence HRS1 protein accumulation, but the P signal does not affect its mRNA accumulation and NO3−response. (a) HRS1–GFP protein accumulation is induced in response to 1 mM NO3−treatment. (b) HRS1–GFP protein accumulation is affected by P provision; 48 h P starvation (reported by IPS1 sentinel regulation) does not affect HRS1 (endogenous gene), HHO1, and HRS1:GFP mRNA accumulation. (c) Rapid NO3−transcriptional activation of HRS1 and subsequent protein accumulation is maintained regardless P provision. Different NO3−levels induce: (i) HRS1–GFP protein accumulation in roots of 48-h P starved plants and (ii) HRS1 transcript accumulation in plant roots grown (14 days) on P varying media. Values are means±s.e.m. (n=3). Figure 4: P and NO 3 − provisions influence HRS1 protein accumulation, but the P signal does not affect its mRNA accumulation and NO 3 − response. ( a ) HRS1–GFP protein accumulation is induced in response to 1 mM NO 3 − treatment. ( b ) HRS1–GFP protein accumulation is affected by P provision; 48 h P starvation (reported by IPS1 sentinel regulation) does not affect HRS1 (endogenous gene), HHO1, and HRS1:GFP mRNA accumulation. ( c ) Rapid NO 3 − transcriptional activation of HRS1 and subsequent protein accumulation is maintained regardless P provision. Different NO 3 − levels induce: (i) HRS1–GFP protein accumulation in roots of 48-h P starved plants and (ii) HRS1 transcript accumulation in plant roots grown (14 days) on P varying media. Values are means±s.e.m. ( n =3). 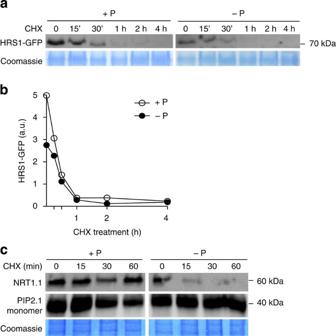Figure 5: P provision affects HRS1 and NRT1.1 protein stability. (a) CHX (100 μM) treatment affects HRS1–GFP accumulation differentially in +P and –P conditions. (b) Quantification of immunoblot signal. (c) P starvation accelerates the protein degradation rate of the nitrate transporter/sensor NRT1.1, but not the aquaporin PIP2.1 (used as non-nitrate-inducible control). Full size image Figure 5: P provision affects HRS1 and NRT1.1 protein stability. ( a ) CHX (100 μM) treatment affects HRS1–GFP accumulation differentially in +P and –P conditions. ( b ) Quantification of immunoblot signal. ( c ) P starvation accelerates the protein degradation rate of the nitrate transporter/sensor NRT1.1, but not the aquaporin PIP2.1 (used as non-nitrate-inducible control). Full size image Genome-wide effect of HRS1 and HHO1 on gene expression To better document the in planta effects from the modification of the HRS1/HHO1 TFs, plantlets (Col, hrs1;hho1 , HRS1-OE and HHO1-OE) were grown in −P/+NO 3 − conditions for 6 days in three independent experiments. Whole roots ( Fig. 6a ) were harvested to measure the effect of these HRS1/HHO1 genetic modifications using last generation Affymetrix chips (Arabidopsis gene1.1ST array, Supplementary Data 2 ). Analysis was performed as previously described in refs 43 , 44 (for details see Methods). Analysis of variance (ANOVA) followed by a post hoc Tukey test yielded 1,125 HRS1/HHO1-regulated probes corresponding to 969 unambiguous genes. A clustering analysis helped to understand the dominant mode of regulation triggered by the mutation or the overexpression of HRS1 and HHO1 ( Fig. 6b ). Among these 969 HRS1/HHO1-regulated genes, 22 genes have been identified to be direct HRS1 targets based on the TARGET approach (11 upregulated and 11 downregulated, Supplementary Data 1 ). This relatively low number is however higher than one would expect by chance (Monte Carlo test P value<0.05). Among these HRS1 direct targets is NRT1.1 , which is found in cluster #8. Since we have shown that NRT1.1 is a key regulator of HRS1 primary NO 3 − induction ( Fig. 1e ), this demonstrates a potential feedback mechanism of HRS1 on its own regulator, as is often found in regulatory networks. The 969 HRS1/HHO1-regulated genes have been subjected to GO enrichment analysis by the agriGO web site [39] followed by a REVIGO analysis to reduce and summarize the number of GO terms detected [45] . Interestingly, this analysis demonstrates that ‘ phosphorus metabolism ’, ‘ hormone metabolism ’, ‘ starch metabolism ’, ‘ developmental process ’, ‘ cellular nitrogen compound metabolism ’, ‘ post-embryonic development ’, ‘ response to red light ’ and ‘ response to abiotic stimulus ’ are (among others; Supplementary Fig. 6 ) enriched in this list. This demonstrates that (i) HRS1/HHO1 indeed affect the processes that have been predicted by the cell-based TARGET system approach ( Fig. 1g ; Supplementary Fig. 6 ), and (ii) that HRS1/HHO1 may have other functions, as the one described herein, some of which that was predicted by other studies (refs 35 , 46 and discussed below). 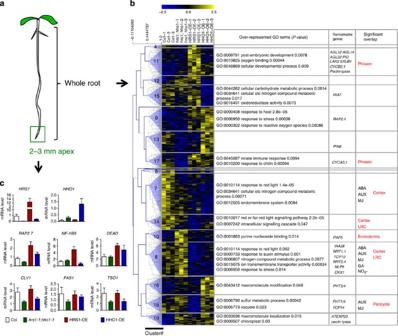Figure 6: Probing the effect of HRS1 and HHO1 mutations and overexpressions in −P-deficient root transcriptome. (a) Six-day-old plantlets were grown on −P/+NO3−conditions (b) or on +P/+NO3−media and then transferred 2 days to −P/+NO3−conditions (c). (b) Clustering of the 969 HRS1-regulated genes from whole roots of plantlets grown on −P/+NO3−media. For each cluster, a selection of over-represented GO terms is given, as well as remarkable genes belonging to the cluster. Clusters overlap with NO3−(ref.31); hormonal59responsive genes or root cell type-specific markers50have been measured using the GeneSect algorithm22. Significant overlaps (Pvalue<0.05) are reported in the third column. (c) Reverse transcription qPCR analysis on selected HRS1 direct targets on RNA extracted from 2- to 3-mm sections of the root apex in a transfer experiment. Values are means±s.e.m. (n=3). Residual HHO1 expression in the mutant is explained inSupplementary Fig. 2. Figure 6: Probing the effect of HRS1 and HHO1 mutations and overexpressions in −P-deficient root transcriptome. ( a ) Six-day-old plantlets were grown on −P/+NO 3 − conditions ( b ) or on +P/+NO 3 − media and then transferred 2 days to −P/+NO 3 − conditions ( c ). ( b ) Clustering of the 969 HRS1-regulated genes from whole roots of plantlets grown on −P/+NO 3 − media. For each cluster, a selection of over-represented GO terms is given, as well as remarkable genes belonging to the cluster. Clusters overlap with NO 3 − (ref. 31 ); hormonal [59] responsive genes or root cell type-specific markers [50] have been measured using the GeneSect algorithm [22] . Significant overlaps ( P value<0.05) are reported in the third column. ( c ) Reverse transcription qPCR analysis on selected HRS1 direct targets on RNA extracted from 2- to 3-mm sections of the root apex in a transfer experiment. Values are means±s.e.m. ( n =3). Residual HHO1 expression in the mutant is explained in Supplementary Fig. 2 . Full size image To obtain further insights into the altered gene responses triggered by altered expression of HRS1/HHO1, a clustering analysis uncovered 19 clusters of mis-regulated genes ( Supplementary Data 2 ). The overall analysis of the 19 clusters demonstrates that even if HRS1 and HHO1 seem to play redundant roles in the control of primary root growth ( Fig. 2 ), they may control at the same time the same set of genes (such as in cluster #9,17,7,14,10,8) or different genes (such as in clusters #4,11,12,15,13,16). AgriGO was then used to determine the molecular coherence of these HRS1/HHO1-regulated gene clusters into potential biomodules (that is, co-regulated genes having a particular function [47] ). Interestingly, in the clusters for which HRS1 and HHO1 have a coherent effect on gene regulation (control the same set of genes), the GO terms are related to ‘ stress responsiveness ’ and ‘ response to reactive oxygen species (ROS)’. Moreover, it seems that HRS1 overexpression is the one that triggers the most regulation on genes responsible for growth control (that is, cluster #11). Taken together, this could suggest that HRS1 and HHO1 play redundant functions due to their phylogenetic proximity, but might control different set of genes depending on the genomic context. However, since the two TFs converge towards the control of ROS signalling-related genes, and that ROS have recently been shown to be involved in the control of primary root meristematic activity [48] or cell size [49] , it is tempting to propose that such a mechanism could be downstream of HRS1/HHO1 influence. It is however important to note that UPB1 does not belong to the 969 HRS1/HHO1-regulated genes based on whole-root transcriptome studies. These hypotheses will need further experiments to be fully validated. One hypothesis related to the modularity of the HRS1 versus HHO1 effect is that they can affect different genes according to the possible tissue context. To document this possibility, the different HRS1/HHO1-controlled gene clusters were overlapped to a set of genes defined as markers of different root cell layers [50] . Interestingly, clusters #11,7,17,14,10,8,18 appear to significantly ( P value<0.05, Monte Carlo test named GeneSect [22] ) overlap with cell type-specific markers (third column, Fig. 6b ). Thus, since the transcriptome is performed at the whole-root level, this overlap may show that some clustering properties are related to different activities of the two TFs in different cell types. Again, this will need to be fully validated by following further experimental studies. The most striking cluster of this analysis is #8. Indeed, it gathers genes being more highly expressed in the double hrs1-1;hho1-1 mutant and repressed by HRS1 or HHO1 overexpression ( Fig. 6b ). Interestingly, this cluster comprises genes known to be responsive to NO 3 − (including NRT1.1 and NRT2.4 , among others) and hormones. Indeed, ‘ response to auxin stimulus ’ is also an over-represented GO term in this gene cluster. This observation opens perspectives concerning the role of auxin signalling in the control of root developmental mechanisms that could explain the effect of HRS1 and HHO1 in −P conditions. To consolidate the fact that HRS1 binds cis -elements of six genes that are found to be direct targets of HRS1, which are activated in the cell-based system ( Figs 1 and 3 ), we wondered why these genes are not found in the 969 HRS1-regulated genes detected in whole roots? Since the P effect is very much localized to the root apex, and likely not affected by the whole-plant P status (according to transfer experiments Supplementary Fig. 3 ), we hypothesized that the regulation by P may be restricted to the most apical part of the root. To validate this hypothesis, we performed transfer experiments from +P/+N to −P/+N media. The tip of the primary root (2–3 mm) was harvested from the WT, hrs1-1;hho1-1 double mutant and overexpressors and RNA used for qPCR experiments. This revealed that RAP2.7 , NF-YB5 and the DEAD helicase are indeed regulated by HRS1 overexpression at the root apex ( Fig. 6c ). Several meristem-related genes ( CLV1 , FAS1 and TSO1 ), defined as direct targets by the cell-based TARGET system ( Supplementary Data 1 ), were also measured and displayed misregulation in the hrs1;hho1 double mutant, but with no effect of the TF overexpression ( Fig. 6c ). This demonstrates that these genes may be indeed under the direct influence of HRS1 in plants, and are potential candidates controlling meristematic activity together with the previously evoked pathways that include auxin and ROS signalling (refers to clusters #8 and #9,15,11, respectively, Fig. 6b ). To decipher the different regulatory pathways below the action of the genes known to sensitize primary root to local P deficiency, it will be important to confront whole-genome expression reprogramming induced by lpr1/2 (ref. 8 ), pdr2 (ref. 9 ) and hrs1;hho1 to define whether these regulatory modules share common signalling pathways. Further, reverse genetic studies will also be needed to validate that the potential regulators of meristematic activity such as CLV1 , FAS1 , TSO1, RAP2.7 or NF-YB5 are indeed a part of the HRS1/HHO1-mediated response. Finally, we believe that this transcriptomic analysis provides an important proxy towards understanding the other roles of HRS1 in plants. Indeed, it has been shown to be controlling germination [51] , or to confer drought or salt stress tolerance [52] . Again the general functions regulated by HRS1 such as ‘ ROS signalling ’, as well the important overlap with ABA responsive genes are important keys to understand the underlying mechanisms behind the previously reported phenotypes. As we take together the above observations, we propose the model described in Fig. 7 . HRS1 is under a dual regulation: (i) a NO 3 − -induced (NRT1.1/CHL1 NLP7 dependent) transcriptional control, and (ii) a Pi-regulated post-transcriptional control. In response to these two signals, HRS1 controls primary root growth through possibly: (i) its action on two independent CREs contained in promoters of activated genes; and (ii) its effect on pathways such as ROS or Auxin signalling. These two possibilities are not exclusive. Our observations can, to some extent, be related to the recent work of Kellermeier et al. [53] , which makes a clear demonstration that nutrient signalling interaction is rather a general rule than an exception. 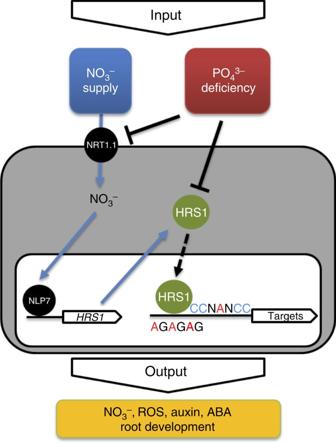Figure 7: Proposed model: NO3−and P limitation signals are integrated by the control of HRS1 at the transcriptional and post-transcriptional level, respectively. On NO3−treatment, the NRT1.1 and NLP7 regulatory module induces rapid HRS1 transcript and protein accumulation. The prolonged P deficiency condition negatively affects the accumulation of HRS1 and modifies its regulatory activity. Furthermore, the P limitation signal seems to control the NO3−sensor (NRT1.1) protein half-life. This delineates a working model to understand several points of NO3−and PO43−signal interactions via the HRS1 pathway. Figure 7: Proposed model: NO 3 − and P limitation signals are integrated by the control of HRS1 at the transcriptional and post-transcriptional level, respectively. On NO 3 − treatment, the NRT1.1 and NLP7 regulatory module induces rapid HRS1 transcript and protein accumulation. The prolonged P deficiency condition negatively affects the accumulation of HRS1 and modifies its regulatory activity. Furthermore, the P limitation signal seems to control the NO 3 − sensor (NRT1.1) protein half-life. This delineates a working model to understand several points of NO 3 − and PO 4 3− signal interactions via the HRS1 pathway. Full size image Our work provides a potential mechanism for understanding how the two key plant mineral nutrients (PO 4 3− and NO 3 − ) interact to control root growth, an issue of global importance, since nitrogen and phosphorus are the two most widely used fertilizers worldwide that maintain plant growth and production. For instance, a recent work by Delgado-Baquerizo et al. showed that at the ecological level, drying lands might impact markedly nitrogen and phosphorus ratios available for plants, thus jeopardizing food production worldwide [54] . The molecular events, mediated by HRS1 and HHO1 in plants, that integrate two mineral-related signalling pathways are part of the fundamental knowledge needed to tackle such key environmental challenge in a global warming context. Plant material All A. thaliana plants were in the Columbia background. Mutant hrs1-1 (SALK_067074), hho1-1 (SAIL_28_D03) and mutant chl1-12 (Salk_034596) were obtained from ABRC seeds stock center. The hrs1-1;hho1-1 double mutant has been obtained by crossing. Despite the presence of a highly accumulated chimeric RNA in the hho1-1 line (characterized in Supplementary Fig. 2c ), the production of a full-length gene product is knocked out ( Supplementary Fig. 2b ). The promoter gene GFP lines for tissue localization were obtained by cloning HRS1 and HHO1 from genomic sequences, bringing respectively the 3- and 2.5-kb upstream promoter region and the gene, into pMDC107 Gateway-compatible vector. Overexpressor lines were obtained by cloning HRS1- and HHO1-coding sequences into pMDC32 Gateway-compatible vector [55] , using primers listed in Supplementary Data 1 . The constructs were transferred to Agrobacterium tumefaciens strain GV3101 and used for the Arabidopsis transformation by the floral dip method [56] . Transgenic plants were selected by antibiotic resistance and T3 homozygote descendants were used for analysis. Growth conditions and treatments For NO 3 − treatment experiment, plants were grown in sterile hydroponic conditions as described in [22] ref. 22. Hydroponic media consisted of MS basal salt medium containing no nitrate and supplemented with 3 mM sucrose, 0.5 mM ammonium succinate, MES buffered at pH 5.7 (0.5 g l −1 ). Plants were grown for 15 days in day/night cycles (16/8 h; 65 μmol photons m −2 s −1 ) at 22 °C. Plants were transferred to an equivalent fresh nitrogen-free medium for 24 h and then treated with nitrogen as 1 mM KNO 3 or 1 mM KCl, as mock treatment. Roots were sampled at different time points after the treatment and immediately frozen in liquid nitrogen. For P starvation experiments, Col-0 and hrs1-1;hho1-1 seeds were sown on the surface of solid media consisting of MS basal salt medium nitrogen and phosphorous-free supplemented with KNO 3 at different concentrations (0.05, 0.5, 1 and 2.5 mM), 0.5 mM KH 2 PO 4 for P-sufficient condition, 3 mM sucrose, MES (0.5 g l −1 ) and 0.8% (w/v) agarose. Different volumes of 1 mM KCl solution were added to the media to keep the K + concentration constant among different conditions. Plants were grown vertically for 9 days in day/night cycles (16/8 h; 90 μmol photons m −2 s −1 ) at 22 °C. For P starvation experiments in liquid media, plants were grown for 15 days in sterile hydroponics conditions, in MS media containing 5 mM KNO 3 and 1 mM KH 2 PO 4 . Plants were transferred towards an equivalent KH 2 PO 4 -free fresh medium (−P) or 1 mM KH 2 PO 4 media (+P) for 48 h. For half-life experiment, CHX was used at 100 μM. All growth and gene expression experiments are supported by at least three independent experiments. Root growth measurements Beginning 2 days after seed sowing, two Petri dishes per condition (that is, at least 30 plants) were scanned every day at 400 d.p.i. Root length was measured using Optimas 6.1 software and statistical differences between genotypes were calculated using Student’s t -test. Real-time qPCR analysis Total RNA was isolated from Arabidopsis roots and shoots using TriReagent (Molecular Research center Inc.) and digested with DNAseI (Sigma-Aldrich, St Louis, USA). Total RNAs were then reverse transcribed to one-strand complementary DNA using Thermo script RT (Invitrogen) according to the manufacturer’s protocol. Gene expression was determined by reverse transcription qPCR (LightCycler 480; Roche Diagnostics, Basel, Switzerland) using gene-specific primers (listed in Supplementary Data 1 ) and LightCycler 480 SYBR Green I Master mix (Roche, IN, USA). Expression levels of tested genes were normalized to expression levels of the actin and clathrin genes. TF perturbation assays in the TARGET system The TARGET procedure has been performed as previously described in Bargmann et al. [36] Protoplasts were treated with 35 μM CHX and 10 μM DEX. The red fluorescent protein was used as marker selection for fluorescent-activated cell sorting of successfully transformed protoplasts. One milimolar NO 3 − was maintained during the whole procedure. RNA was extracted and amplified for hybridization with ATH1 Affymetrix chips. Data were analysed with R. Mas5 normalized data were extracted and analysed by a t -test procedure for DEX response ( P value<0.05, fold regulation>2 × , corresponding to a false discovery rate<0.1). Microscopy Col-0, pHRS1:HRS1:GFP and pHHO1:HHO1:GFP seedlings were grown on half-strength MS media for 8 days. The same liquid media was used for mounting plantlets during the image capture. Fluorescence imaging was performed using the Olympus BX61 microscope. Samples were excited at 470 nm and emission was collected between 500 and 535 nm. Confocal images were performed with a Zeiss LSM510 Meta laser scanning microscope. Root cell walls were stained with propidium iodine 10 μg ml −1 (Sigma) and nucleus with 4,6-diamidino-2-phenylindole 1 μg ml −1 (Sigma). Three-dimensional root reconstructions were obtained from confocal Z series using the Imaris software. Semantic gene enrichment analysis To identify the most represented gene functions for each gene list, the gene descriptions of targets were retrieved from TAIR web site ( http://www.arabidopsis.org/index.jsp ) and the list was analysed using a software developed in R ( http://www.r-project.org/ ). Briefly, given the list of 551 HRS1 up-/downregulated genes, the software counts the occurrence of each term of the description and compares it with the occurrence of the same term in 1,000 random lists of the same size. Results are presented as a cloud of words, whose colour and size are correlated to their occurrence. Phylogenetic analysis The phylogeny reconstruction was inferred by using the maximum likelihood method. The 40 sequences coding for G2-like proteins were retrieved from the AGRIS (Arabidopsis Gene Regulatory Information Server; http://arabidopsis.med.ohio-state.edu/ ) database. The bootstrap values were obtained based on 500 replicates. Evolutionary analysis was conducted in MEGA5 software [57] . Expression and purification of recombinant GST-HRS1 protein HRS1 coding sequence CDS was first cloned in pDONR207, using the primers listed in Supplementary Data 1 and then transferred to pDEST15 vector (Invitrogen) by LR reaction following the manufacturer’s instructions. The GST-HRS1 fusion protein was expressed in Escherichia coli Rosetta 2(DE3)pLysS (Novagen, Darmstadt, Germany) cells after induction with 1 mM isopropyl-β- D -thiogalactoside for 16 h at 22 °C. Bacteria were harvested, suspended in PBS buffer containing lysozyme from chicken egg white (Sigma) and complete protease inhibitor cocktail (Roche) and sonicated. The protein extract was purified on glutathione sepharose beads (GE Healthcare, Freiburg, Germany), eluted with 10 mM reduced glutathione (Sigma), 50 mM Tris buffer and dialysed overnight in 150 mM NaCl, 50 mM HEPES, pH 7.4 buffer. EMSA Purified GST-HRS1 recombinant protein was used to determine DNA binding by EMSA. Single-stranded DNA oligonucleotides (listed in Supplementary Data 1 ) were biotin labelled using the Biotin 3′ End DNA Labelling Kit (Thermo Scientific) and complementary pairs were annealed to make double-stranded DNA probes. The binding of recombinant protein (50 ng) to the biotin-labelled probes (20 fmol) was carried out in a reaction mixture containing 10 mM Tris, 50 mM KCl, 1 mM DTT, pH 7.5, 2.5% glycerol, 5 mM MgCl 2 , 1 μg poly (deoxyinosinic–deoxycytidylic) and 0.05% NP-40. After incubation at 22 °C for 30 min, the protein–probe mixture was separated in a 4% polyacrylamide native gel and transferred to a Biodyne B Nylon membrane by capillary action in 20 × SSC buffer overnight (Thermo Scientific). After ultraviolet crosslinking (254 nm) for 90 s at 120 mJ·cm −2 , the migration of biotin-labelled probes was detected using streptavidin horseradish peroxidase conjugates in the Chemioluminescent Nucleic Acid Detection Module (Thermo Scientific) and exposed to X-ray film. As a negative control, we tested that the GST tag has no affinity for HRS1-related CREs ( Supplementary Fig. 5 ). Protein extraction and immunoblot analysis Roots were sampled and frozen in liquid nitrogen. Total proteins were obtained using the Plant Total Protein Extraction Kit (Sigma) and quantified with the Pierce 660 nm Protein Assay using a BSA standard curve. Membrane proteins were obtained by disrupting roots in a buffer containing a plant anti-protease cocktail (Sigma-Aldrich) and anti-phosphatases (30 mM glycerophosphate, 5 mM molybdate and 10 mM NaF). The whole-membrane fraction was then isolated by centrifugation (100,000 g , 4 h) on a 55% sucrose cushion. Immunoblot analysis was performed on 40–50 μg of proteins using anti-GFP–HRP 1:2,500 (Miltenyi Biotec, 130-091-833), anti-NRT1.1 1:5,000 (AS12 2611, Agrisera) and anti-PIP2.1 1:5,000 (ref. 58 ). Coomassie Brilliant Blue staining of blots was used to control the protein levels after electrotransfer. Uncropped versions of the blots are provided in Supplementary Figs 7 and 8 . Band intensity quantification was performed using a chemioluminiescent image analyser LAS3000 (Fujifilm) and ImageGauge (Fujifilm) software. Transcriptome analysis The transcriptome analysis was performed using the GeneChip Whole Transcript (WT) Expression Array following the manufacturer’s protocol. Total RNA was isolated from 6-day-old roots grown on media containing 2.5 mM KNO 3 and no PO 4 3− (three independent experiments). RNA integrity numbers were checked by microfluidic analysis in an Agilent 2100 Bioanalyzer. Complementary DNAs were prepared from 150 ng of total RNA following the WT Plus Reagent Kit protocol, hybridized on Affymetrix Array Strip and processed on the GeneAtlas System. Data set analysis was performed with R. A one-way ANOVA model was applied (four levels: Col, hrs1-1;hho1-1 , HRS1-OE and HHO1-OE) followed by a post hoc Tukey test (R functions aov() and TukeyHSD() ). Any probe having a significant P value<0.05 for the ANOVA or the Tukey test was kept for further analysis. Clustering analysis was performed with MeV software (distance, Pearson correlation). Accession codes: Microarray data associated with this study has been deposited in NCBI GEO database under the accession code GSE64352 . How to cite this article: Medici, A. et al. AtNIGT1/HRS1 integrates nitrate and phosphate signals at the Arabidopsis root tip. Nat. Commun. 6:6274 doi: 10.1038/ncomms7274 (2015).